Domain topology and domain switching kinetics in a hybrid improper ferroelectric Charged polar interfaces such as charged ferroelectric walls or heterostructured interfaces of ZnO/(Zn,Mg)O and LaAlO 3 /SrTiO 3 , across which the normal component of electric polarization changes suddenly, can host large two-dimensional conduction. Charged ferroelectric walls, which are energetically unfavourable in general, were found to be mysteriously abundant in hybrid improper ferroelectric (Ca,Sr) 3 Ti 2 O 7 crystals. From the exploration of antiphase boundaries in bilayer-perovskites, here we discover that each of four polarization-direction states is degenerate with two antiphase domains, and these eight structural variants form a Z 4 × Z 2 domain structure with Z 3 vortices and five distinct types of domain walls, whose topology is directly relevant to the presence of abundant charged walls. We also discover a zipper-like nature of antiphase boundaries, which are the reversible creation/annihilation centres of pairs of two types of ferroelectric walls (and also Z 3 -vortex pairs) in 90° and 180° polarization switching. Our results demonstrate the unexpectedly rich nature of hybrid improper ferroelectricity. Over the last decade, two-dimensional (2D) conduction in heterostructured interfaces with polar discontinuity [1] , [2] or compositionally homogeneous charged interfaces such as charged ferroelectric domain walls (FE DWs) [3] , [4] , [5] , [6] , [7] , [8] , [9] , [10] has attracted enormous attention for emergent phenomena and new material functionalities. However, undesirable chemical/structural complexity such as ionic diffusion, oxygen vacancies or structural/strain variations near the interface results in equivocal interpretation of the origin of 2D conduction [11] , [12] , [13] . In parallel, significant efforts have been launched to investigate the 2D conduction at charged FE DWs, which are well defined at the atomic scale. The conducting FE DWs were observed in chemically homogeneous thin films, for example, Pb[Zr x Ti 1-x ]O 3 (ref. 14 ), BiFeO 3 (ref. 10 ) and Bi 0.9 La 0.1 FeO 3 /SrRuO 3 heterostructure [9] and bulk single crystals, for example, LiNbO 3 (ref. 4 ), BaTiO 3 (ref. 5 ) and Er(Ho)MnO 3 (refs 6 , 7 ). These conducting FE DWs are intrinsically unstable because of large energy cost [8] , [15] , often pinned by chemical defects [4] and sporadically [5] and artificially created with external voltage [9] . However, charged domain walls (DWs), some of which are highly conducting, were found to be abundant in the hybrid improper FE (Ca,Sr) 3 Ti 2 O 7 (ref. 3 ). Ordering phase transitions in condensed matter can be accompanied by directional variants and antiphase boundaries (APBs). Directional-variants result in domains with different directional order parameters. The role of APBs [16] , [17] on materials functionalities has been well recognized [18] , [19] , [20] , [21] , [22] . In particular, the discovery of strong interaction or interlocking nature of APBs with ferroic orders in diverse functional materials opens new grounds for material research. Examples include the ferromagnetic coupling in Heusler alloys [23] , the reduced spin polarization in half-metal magnetites [24] , the duality nature of DWs and topological defects in hexagonal manganites [25] , FE APBs in a nonpolar matrix [16] and conducting and ferromagnetic walls of antiferromagnetic domains in pyrochlore iridates [26] . Hybrid improper ferroelectricity (HIF), a phenomenon involving polarization induced by a hybridization of two non-polar lattice instabilities, offers great promise towards the realization of room-temperature multiferroism [27] , [28] , [29] , [30] , [31] . The key idea is to design new materials in which ferroelectricity and (anti)ferromagnetism can be coupled by the same lattice instability, therefore providing an indirect but strong coupling between polarization and magnetism [27] , [28] , [29] , [31] , [32] . Examples of compounds with HIF include the double-layered Ruddlesden-Popper perovskites with the chemical formula of A 3 B 2 O 7 ( Fig. 1 , A 2+ =alkali metal; B 4+ =transition metal) [3] , [27] , [32] . Unexpectedly, charged FE DWs, some of which are highly conducting, were also found to be mysteriously abundant in the recently discovered Ruddlesden-Popper-type HIF (Ca,Sr) 3 Ti 2 O 7 crystals [3] . 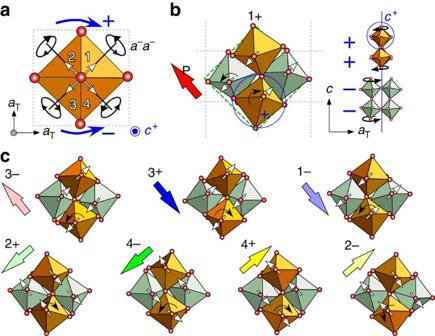Figure 1: Structural illustrations of the eight ferroelectric domains in A3B2O7. (a) An in-plane BO6octahedral constituent with tilting along the <110>Tdirections and rotation around the [001]Tdirection. Plus (+) and minus (−) represent clockwise and anticlockwise rotations. White arrows indicate the displaced directions (1stto 4thquadrants) of the apical oxygen of the BO6octahedron due to octahedral tilting. The red spheres represents O ions. (b) The 1+ domain state. The red arrow indicates the polarization direction. The grey dotted lines depict the basic tetragonal framework constructed by B-site ions and the green dashed rectangle depicts the orthorhombic cell. The cross-sectional structure includes two bi-layers formed by orange and light green corner-sharing BO6octahedra. Each domain state can be unambiguously identified by naming the distortions of a given octahedron (blue-circled) as the five adjacent octahedra in each bi-layer are constrained to tilt and to rotate in opposite senses, and also the overall crystallographic symmetry (A21am) determines the distortions in the adjacent bi-layers. (c) The in-plane structural models of the 1−, 2±, 3± and 4± domain states. Switching of the octahedral tilting pattern is involved between two domain states in, for example, 1+ versus 3+, 1− versus 3−, 2+ versus 4+ and 2− versus 4−, and switching of the octahedral rotation pattern is required between 1+ versus 1−, 2+ versus 2−, 3+ versus 3− and 4− versus 4+. Antiphase domain relations can be found between two domain states in, for example, 1+ versus 3−, 1− versus 3+, 2+ versus 4− and 2− versus 4+. The corresponding polarization direction in each domain state can be derived readily from our nomenclature; for example, the 1+ domain state accompanies a polarization towards the 2nd quadrant—starting from the 1st quadrant and rotating clockwise (+) to the 4th quadrant that results in the nearest A-site cation (and polarization) being displaced in the opposite direction to the 2ndquadrant. Note that the net in-plane dipole moment (Γ5−) is caused by this A-site-cation displacement. Figure 1: Structural illustrations of the eight ferroelectric domains in A 3 B 2 O 7 . ( a ) An in-plane BO 6 octahedral constituent with tilting along the <110> T directions and rotation around the [001] T direction. Plus (+) and minus (−) represent clockwise and anticlockwise rotations. White arrows indicate the displaced directions (1 st to 4 th quadrants) of the apical oxygen of the BO 6 octahedron due to octahedral tilting. The red spheres represents O ions. ( b ) The 1+ domain state. The red arrow indicates the polarization direction. The grey dotted lines depict the basic tetragonal framework constructed by B-site ions and the green dashed rectangle depicts the orthorhombic cell. The cross-sectional structure includes two bi-layers formed by orange and light green corner-sharing BO 6 octahedra. Each domain state can be unambiguously identified by naming the distortions of a given octahedron (blue-circled) as the five adjacent octahedra in each bi-layer are constrained to tilt and to rotate in opposite senses, and also the overall crystallographic symmetry ( A2 1 am ) determines the distortions in the adjacent bi-layers. ( c ) The in-plane structural models of the 1−, 2±, 3± and 4± domain states. Switching of the octahedral tilting pattern is involved between two domain states in, for example, 1+ versus 3+, 1− versus 3−, 2+ versus 4+ and 2− versus 4−, and switching of the octahedral rotation pattern is required between 1+ versus 1−, 2+ versus 2−, 3+ versus 3− and 4− versus 4+. Antiphase domain relations can be found between two domain states in, for example, 1+ versus 3−, 1− versus 3+, 2+ versus 4− and 2− versus 4+. The corresponding polarization direction in each domain state can be derived readily from our nomenclature; for example, the 1+ domain state accompanies a polarization towards the 2nd quadrant—starting from the 1st quadrant and rotating clockwise (+) to the 4th quadrant that results in the nearest A-site cation (and polarization) being displaced in the opposite direction to the 2 nd quadrant. Note that the net in-plane dipole moment (Γ 5 − ) is caused by this A-site-cation displacement. Full size image To unveil the origin of these abundant charged FE DWs, we have explored the complete connectivity of DWs in Ca 2.55 Sr 0.45 Ti 2 O 7 (CSTO; FE Tc≈790 K) and Ca 3 Mn 1.9 Ti 0.1 O 7 (CMTO; FE Tc≈360 K) single crystals with in-plane polarization along the pseudo-tetragonal [110] directions [3] , [30] , [33] , particularly with mapping of APBs using transmission electron microscopy (TEM). Note that APBs are invisible in piezoresponse force microscopy (PFM) [34] , which is usually a good method to map out FE domain configurations. Phase-field simulations [35] were also conducted to understand the origin of domain configurations in CMTO and CSTO. Our results reveal that the formation of a unique Z 4 × Z 2 domain topology with Z 3 vortices is responsible for the presence of abundant charged FE DWs in CSTO. In addition, we have also investigated the kinetics associated with polarization switching in CSTO, understanding of which is crucial for developing precise control of conducting FE walls. Z 4 × Z 2 domain structure with eight different states Figure 1a shows two characteristic lattice modes in A 3 B 2 O 7 : First, the BO 6 octahedral in-phase rotations are either clockwise (the sign of the rotation is +) or anticlockwise (−) about a [001] T direction (denoted as a 0 a 0 c + in the Glazer notation [36] or the X 2 + mode), and second, the BO 6 octahedral tilting occurs about two <110> T axes, that is, apical oxygen-motions displace towards the 1st to 4th quadrants (denoted as a − a − c 0 or the X 3 − mode) with respect to the high-symmetry tetragonal I4/mmm (T, space group #139) structure. Below the phase transition, the X 3 − mode adopts one of the four tilts (1–4) accompanying the X 2 + mode with + or − rotations into a combined distortion pattern of a − a − c + having eight degenerate states, which we label as 1±, 2±, 3± and 4± (the complete structures are shown in Fig. 1b,c ). Figure 1b shows the 1+ state projected along the [001] T and [010] T directions. For example, the apical oxygen of the blue-circled octahedron moves towards the 1 st quadrant (white arrow) with a clockwise rotation (black curved arrow) to form a 1+ state. A trilinear coupling among the X 2 + mode, X 3 − mode and the polar Γ 5 − mode (A-site displacement) yields four FE polarizations parallel or antiparallel to the two <110> T tilting axes [3] , [27] . We emphasize that each polarization direction is associated with two degenerate states, for example, the 1+ and 3− polarizations point in the same direction (red and light-red arrows in Fig. 1b,c ), a consequence of both nonpolar order parameters (X 3 − and X 2 + ) changing signs. These four polarization directional variants with twofold degeneracy form the basis of the Z 4 × Z 2 domain structures in the HIF A 3 B 2 O 7 . 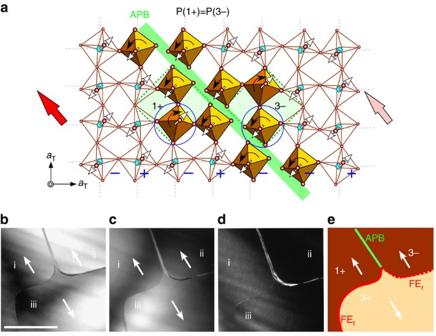Figure 2: Antiphase boundary (APB) in a CSTO crystal. (a) The local distortions near an [110]T-oriented APB (green line) between the 1+ and 3− states, which are identical in polarization direction but differ in structure with respect to rotation (black curved arrows) and tilting (white arrows) by 180°. (b) Aab-plane DF-TEM image taken using superlatticeg1+=3/2(1, 1, 0)Tspot. (c) A DF-TEM image taken using superlatticeg1−=3/2(−1, −1, 0)Tspot. A reversed contrast inb,cdemonstrates the characteristic of 180°-type FE domains. (d) A DF-TEM image taken usingg1−spot at a large tilting angle to tune contrast by enhancing excitation error. A clear boundary interference fringe can then be observed between domains ii and iii, implying an inclined nature and a strong strain gradient expected in rotation-driven FErDWs. (e) The schematic domain configuration obtained fromb–ddemonstrates a typical Z3vortex pattern within a FA domain, composed of three 180°-FE domains and three DWs: FEr(red-dotted), FEt(red-solid) DWs and APB (green-solid). White arrows denote the polarization directions in FE domains. Scale bar, 500 nm. Figure 2a shows a structural model of a APB (green line) between the 1+ and 3− states, at which the orthorhombic unit cells labelled by green dotted lines illustrate the discontinuation of octahedral tilting (white arrows) and rotation (+ and −) at the wall. APBs might exist in A 3 B 2 O 7 , but behave hidden in the PFM images as the two domains give the same piezo-response [3] . Figure 2: Antiphase boundary (APB) in a CSTO crystal. ( a ) The local distortions near an [110] T -oriented APB (green line) between the 1+ and 3− states, which are identical in polarization direction but differ in structure with respect to rotation (black curved arrows) and tilting (white arrows) by 180°. ( b ) A ab -plane DF-TEM image taken using superlattice g 1 + =3/2(1, 1, 0) T spot. ( c ) A DF-TEM image taken using superlattice g 1 − =3/2(−1, −1, 0) T spot. A reversed contrast in b , c demonstrates the characteristic of 180°-type FE domains. ( d ) A DF-TEM image taken using g 1 − spot at a large tilting angle to tune contrast by enhancing excitation error. A clear boundary interference fringe can then be observed between domains ii and iii, implying an inclined nature and a strong strain gradient expected in rotation-driven FE r DWs. ( e ) The schematic domain configuration obtained from b – d demonstrates a typical Z 3 vortex pattern within a FA domain, composed of three 180°-FE domains and three DWs: FE r (red-dotted), FE t (red-solid) DWs and APB (green-solid). White arrows denote the polarization directions in FE domains. Scale bar, 500 nm. Full size image Z 3 vortices in the Z 4 × Z 2 domain structures of (Ca,Sr) 3 Ti 2 O 7 Polarized optical microscope images on CSTO and CMTO crystals both clearly exhibit orthorhombic twins, that is, orthorhombically distorted ferroelastic (FA) domains. In addition, in-plane PFM studies show the intriguing FE domains comprising abundant meandering head-to-head and tail-to-tail charged DWs [3] ( Supplementary Fig. 1 ). Compared with PFM, dark-field TEM (DF-TEM) under systematic controlled diffraction conditions allows us to light up domains induced directly by local structural deformations [37] . Figure 2b–d shows a series of DF-TEM images taken along the [001] T direction using superlattice peaks g 1 ± =±3/2(1, 1, 0) T parallel to the polar axis within a single FA domain. Three domains (i–iii) in Fig. 2b–d , in which domains i and ii reveal the same domain contrast but opposite to domain iii in contrast, show the existence of antiphase domains i and ii, and an APB between them. Three FE domains including two antiphase domains merging at one vertex point are well illustrated in Fig. 2b–d . As a sense of rotation along the merging three domains is defined in the phase space (see below), their intersection can be called a Z 3 vortex. Note that the relative polar ±a orth directions can be identified from the related electron diffraction patterns but the absolute polarization direction cannot be. Thus, once the polarization direction is chosen for one domain, then the polarization directions in other domains can be fully assigned without ambiguity. Evidently, the existence of APBs remains unchanged even if the assignment of the polarization direction is reversed. Figure 2e depicts one possible assignment with 1+ and 3− antiphase domains. The APB between these 1+ and 3− domains accompanies the sign change of both rotation and tilting ( Fig. 2a ). The presence of an APB and a Z 3 vortex also suggests the existence of pure rotation ( a 0 a 0 c + )-driven DWs and pure tilting ( a − a − c 0 )-driven DWs. We define a tilting-type FE t DW (rotation-type FE r DW) as the wall between adjacent FE domains having opposite a − a − c 0 tilting ( a 0 a 0 c + rotation) but identical a 0 a 0 c + rotation ( a − a − c 0 tilting). The structural details of FE t and FE r DWs are shown in Supplementary Figs 2 and 3 . Note that the Z 3 vortex in Fig. 2e consists of three distinct walls: FE r (red-dotted), FE t DWs (red-solid) and APB (green line). 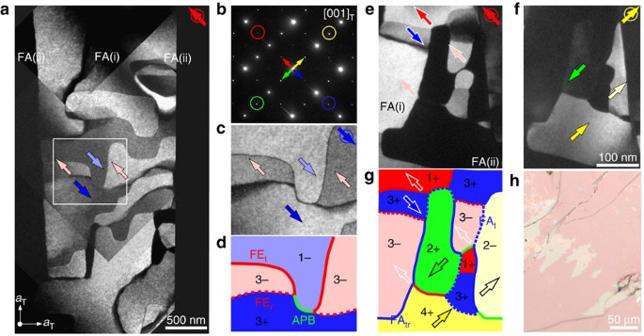Figure 3: The Z3-vortex patterns in Ca2.55Sr0.45Ti2O7and Ca3Mn1.9Ti0.1O7crystals. (a) A 2.2 × 3.9 μm2mosaic of DF-TEM images were taken using the superlatticeg1+spot (red-circled) of domain FA(i) in a CSTO crystal along [001]T. The coloured arrows represent polarization directions within the domain. (b) The electron diffraction pattern was taken by covering regions FA(i) and FA(ii) showing a 90°-crystallographic-twin relation. The red/blue circled spots were contributed from the orthorhombic distortions of the FA(i) region and the green/yellow ones were from the FA(ii) area. The colour-circled spot located in each DF image is the selected superlattice Bragg spot to light up the corresponding domains at a given orientation. (c) A DF-TEM image of the white rectangular box region was taken using the blue circled superlatticeg1−spot. (d) A proposed domain configuration ofc. (e,f) DF-TEM images taken using (e) red circle and (f) yellow circle spots corresponding to superlatticeg1+spots in a CMTO crystal. A Z3-vortex network appears, with three DWs meeting at one point and with irregular shaped FE/FA domains. (g) A proposed domain configuration ofe. Two types of FA DWs, FAt(blue-dotted) and FAtr(blue-solid), were identified. (h) Polarized optical image of a CMTO crystal showing irregular twin (that is, FA) domains in a hundreds micrometre scale. Figure 3a shows a mosaic of DF-TEM images covering three FA (that is, orthorhombic twin; FA(i) and FA(ii)) regions in a CSTO crystal. In the DF-TEM image obtained using orthorhombic superlattice peaks g 1 ± contributed from the FA(i) domain marked by red and blue circles in Fig. 3b , the neighbouring FA(ii) regions exhibit a dark contrast ( Fig. 3a ). Aside from the major contrast between FA(i) and FA(ii), a self-organized Z 3 -vortex network is clearly visible within the FA(i) region. Figure 3c shows a reversed contrast within the white rectangular box taken using a g 1 − spot (blue-circled) and the schematic ( Fig. 3d ) shows a pair of Z 3 vortices is linked by an APB (green line). Boundaries between the 3− (pink) and 3+ (blue) domains form broad contrast walls, identified as FE r DWs (red-dotted lines of Fig. 3d ). By comparing the domain contrasts ( Fig. 3c ), wall features and the neighbouring FA domains obtained from our DF-TEM images, we completely assign all domain states and wall types appearing in Fig. 3a (see the Methods for details). Figure 3: The Z 3 -vortex patterns in Ca 2.55 Sr 0.45 Ti 2 O 7 and Ca 3 Mn 1.9 Ti 0.1 O 7 crystals. ( a ) A 2.2 × 3.9 μm 2 mosaic of DF-TEM images were taken using the superlattice g 1 + spot (red-circled) of domain FA(i) in a CSTO crystal along [001] T . The coloured arrows represent polarization directions within the domain. ( b ) The electron diffraction pattern was taken by covering regions FA(i) and FA(ii) showing a 90°-crystallographic-twin relation. The red/blue circled spots were contributed from the orthorhombic distortions of the FA(i) region and the green/yellow ones were from the FA(ii) area. The colour-circled spot located in each DF image is the selected superlattice Bragg spot to light up the corresponding domains at a given orientation. ( c ) A DF-TEM image of the white rectangular box region was taken using the blue circled superlattice g 1 − spot. ( d ) A proposed domain configuration of c . ( e , f ) DF-TEM images taken using ( e ) red circle and ( f ) yellow circle spots corresponding to superlattice g 1 + spots in a CMTO crystal. A Z 3 -vortex network appears, with three DWs meeting at one point and with irregular shaped FE/FA domains. ( g ) A proposed domain configuration of e . Two types of FA DWs, FA t (blue-dotted) and FA tr (blue-solid), were identified. ( h ) Polarized optical image of a CMTO crystal showing irregular twin (that is, FA) domains in a hundreds micrometre scale. Full size image Domain topology of Ca 3 (Mn,Ti) 2 O 7 We also grew high-quality CMTO single crystals and confirmed the presence of polar domains in the same polar space group ( A2 1 am ) as Ca 3 Ti 2 O 7 at 300 K. Figure 3h shows a polarized optical microscopy image of surprisingly irregular FA DWs on the cleaved (001) T surface, distinct from the prototypical straight FA DWs (that is, orthorhombic twin walls) in CSTO. Our DF-TEM images ( Fig. 3e,f ) demonstrate consistently the presence of irregular twin patterns. The FA(i) domain is excited when the red-circled g 1 + spot was used for imaging ( Fig. 3e ), and it turns to deep-dark contrast when the orthogonal yellow-circled spot was excited ( Fig. 3f ). Inside each FA domain, there exist 180°-type FE domains; for example, bright and grey contrast domains in Fig. 3e,f and Supplementary Fig. 4 . The domain configuration shown in Fig. 3g displays the presence of Z 3 vortices with three domains merging at the vortex cores, which exist within a FA domain, as well as at boundaries between FA domains. Thus, the configuration of Z 3 -vortex domains seems universal in the HIF A 3 B 2 O 7 , despite the existence of eight possible structural variants. Note that there exist two types of FA DWs: ferroelastic tilting DWs (FA t DW) between states in the same rotation, for example, the 1+ and 2+ or 3− and 2− (blue-dotted lines in Fig. 3d and Supplementary Fig. 2 ), and FA tilting+rotation (FA tr ) DWs between, for example, the 2+ and the 3− states (blue lines in Fig. 3d and Supplementary Fig. 2 ). A single tilting of either a − a 0 c 0 or a 0 a − c 0 type may occur at FA t and FA tr DWs (white arrows in Supplementary Fig. 2 ). FA tr DWs seem naturally accompanied with a complete octahedral-rotation frustration at the walls, implying a higher energy of FA tr DWs than that of FA t DWs ( Supplementary Fig. 3 ). Phase-field simulations We also employed the phase-field method (Methods and Tables 1 , 2 , 3 ) [35] to investigate the domain structure of HIF A 3 B 2 O 7 , as shown in Fig. 4a,b . The details of the simulations are given in the Methods. The eight states are represented by different colours. Ca 3 Ti 2 O 7 exhibits straight FA DWs ( Fig. 4a ), consistent with the experimental observation [3] ( Supplementary Fig. 1 ). Across the FA DWs, a dark colour tends to become another dark colour, for example, a red (1+) colour tends to change to a green (2+) colour, rather than to a light green (4−) colour ( Fig. 4a , circle ii). Similarly, two light colours tend to be close with each other across the FA DWs ( Fig. 4a , circle iii). These indicate that the rotation order parameter tends to be unchanged across the FA DWs [38] , which is consistent with the previous discussion on the low energy of FA t , compared with FA tr DWs. Supplementary Fig. 3 shows the oxygen positions of the eight states relative to the tetragonal position. With the assumption that a wall going through a tetragonal-like state with zero polarization costs more energy, the energy hierarchy among the five DWs can be estimated to be FA t ≤FE r ≤FE t ≤FA tr ≤APB. The statistics of DW lengths obtained from phase-filed simulation results give a ratio of FE r :FA t :FE t :APB:FA tr =34:28:28:8:2 in Ca 3 Ti 2 O 7 ( Fig. 4a ) and FA t :FE r :FA tr :FE t :APB=52:22:12:7:7 in Ca 3 Mn 2 O 7 ( Fig. 4b ). A comparably large population of FE t , FE r and FA t walls, especially in Ca 3 Ti 2 O 7 , suggests that APB and FA tr walls belong to the higher energy set than others. Experimentally, within a limited number of DWs that we have observed, CSTO exhibits an 82% population of the lower energy set (FE r , FE t and FA t walls), whereas CMTO shows a 64% population. The low population in CMTO is likely related with the existence of irregular FA domains in CMTO. Note that although an energy hierarchy may exist, we do observe experimentally and theoretically all five kinds of DWs. Table 1 DFT calculated coefficients for the Landau polynomial. Full size table Table 2 DFT calculated elastic stiffness tensor coefficients. Full size table Table 3 Normalized gradient energy coefficients. 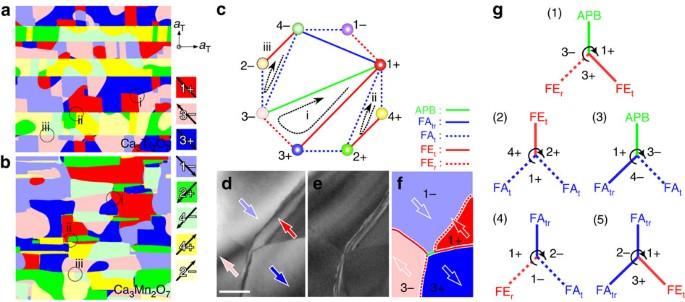Figure 4: Z4× Z2domain with Z3vortices in Ca3Ti2O7and Ca3Mn2O7. (a,b) In-plane domain structures of Ca3Ti2O7and Ca3Mn2O7from phase-field simulations. The eight colours denote the eight domain variants as listed. Z3vortices corresponding to loops i–iii are denoted by black circles in spite of different nature of FA domains in Ca3Ti2O7and Ca3Mn2O7. (c) Schematic of the energy diagram in A3B2O7compounds with eight vertices, representing eight domain variants. Each vertex is connected to seven edges that correspond to one of five types of DWs as shown in the right side. Loops i–iii depict possible vortex domains and domain walls (in fact, Z3vortices). Note that non Z3-type vortex domains corresponding to loops connecting, for example, (1+, 3+, 3−, 1−, 1+) or (1+, 2+, 3+, 3−, 1+) have not been observed experimentally. (d–f) Experimental DF-TEM images demonstrate two Z3vortices at a very short interval of 50 nm in a Ca3Ti2O7crystal. Scale bar, 100 nm. (d) Image was taken under a Friedel’s-pair-breaking condition to reveal 180°-type domain contrast. Polarization directions were shown by white arrows. (e) Image was taken under a larger tilting angle to reveal boundary interference fringes clearly. The width of bent fringes indicates a broad DW interrupting the connection of 1+ (red) and 3− (pink) domains. (f) Image shows a schematic of the corresponding domain configuration. (g) Five possible Z3-vortex configurations derived from the energy diagram. The indicated domain states are examples. Type 1, the only Z3-vortex configuration appearing within a single orthorhombic twin. Type 2, the most common Z3vortex across the orthorhombic twin boundaries. Type 3, Z3vortex accompanying 90° ferroelectric switching at APB. Type 4, Z3vortex accompanying ferroelectric switching in the absence of APB. Type 5, the least favoured Z3vortex with two high energy FAtrwalls. Full size table Figure 4: Z 4 × Z 2 domain with Z 3 vortices in Ca 3 Ti 2 O 7 and Ca 3 Mn 2 O 7 . ( a , b ) In-plane domain structures of Ca 3 Ti 2 O 7 and Ca 3 Mn 2 O 7 from phase-field simulations. The eight colours denote the eight domain variants as listed. Z 3 vortices corresponding to loops i–iii are denoted by black circles in spite of different nature of FA domains in Ca 3 Ti 2 O 7 and Ca 3 Mn 2 O 7 . ( c ) Schematic of the energy diagram in A 3 B 2 O 7 compounds with eight vertices, representing eight domain variants. Each vertex is connected to seven edges that correspond to one of five types of DWs as shown in the right side. Loops i–iii depict possible vortex domains and domain walls (in fact, Z 3 vortices). Note that non Z 3 -type vortex domains corresponding to loops connecting, for example, (1+, 3+, 3−, 1−, 1+) or (1+, 2+, 3+, 3−, 1+) have not been observed experimentally. ( d – f ) Experimental DF-TEM images demonstrate two Z 3 vortices at a very short interval of 50 nm in a Ca 3 Ti 2 O 7 crystal. Scale bar, 100 nm. ( d ) Image was taken under a Friedel’s-pair-breaking condition to reveal 180°-type domain contrast. Polarization directions were shown by white arrows. ( e ) Image was taken under a larger tilting angle to reveal boundary interference fringes clearly. The width of bent fringes indicates a broad DW interrupting the connection of 1+ (red) and 3− (pink) domains. ( f ) Image shows a schematic of the corresponding domain configuration. ( g ) Five possible Z 3 -vortex configurations derived from the energy diagram. The indicated domain states are examples. Type 1, the only Z 3 -vortex configuration appearing within a single orthorhombic twin. Type 2, the most common Z 3 vortex across the orthorhombic twin boundaries. Type 3, Z 3 vortex accompanying 90° ferroelectric switching at APB. Type 4, Z 3 vortex accompanying ferroelectric switching in the absence of APB. Type 5, the least favoured Z 3 vortex with two high energy FA tr walls. Full size image The energy diagram for the HIF A 3 B 2 O 7 such as Fig. 4c can be constructed with all eight states (vertices) and all five kinds of walls (edges connecting two vertices). Note that in Fig. 4c , only a small part of edges are shown, and each vertex is connected to all of the rest vertices through edges in the full energy diagram. The i, ii and iii loops in Fig. 4c correspond to Z 3 vortices in the Fig. 4a,b , respectively. The presence of only Z 3 vortices indicates that the energy difference among five types of DWs is not large, so the lowest-energy vortex defect is always Z 3 -type. Note that if, for example, APB is associated with much higher energy than others, then APB will be fully avoided, and Z 4 -type vortex defects such as 1+/3+/3−/1−/1+ can occur, but we observe only Z 3 -type vortices. In low-magnification TEM images, we sometimes observe vortices looking like Z 4 -type. However, all these likely Z 4 -type vortices turn out to be pairs of closely linked Z 3 vortices with inclined broad DWs, as shown in Fig. 4d–f . The energy diagram ( Fig. 4c ) is, in fact, a hyper-tetrahedron in seven dimensions, which has eight vertices and only triangular faces. Each triangular face in this hyper-tetrahedron corresponds to a Z 3 vortex. All possible configurations of Z 3 vortex derived from the energy diagram ( Fig. 4c ) are shown in Fig. 4g and have been observed experimentally. The configuration of Z 3 vortex domains seems universally adopted in HIF A 3 B 2 O 7 compounds. Note that FA DWs in Ca 3 Ti 2 O 7 , nucleated from a high-temperature tetragonal phase ( I4/mmm ) [33] , [39] , tend to be straight, whereas FA DWs in Ca 3 Mn 2 O 7 , nucleated from the Acaa (space group #68) phase [30] below ∼ 360 K, are irregular ( Supplementary Fig 4 ). A phase-field simulation for the nucleation and growth of the FE A2 1 am domains from the Acaa matrix is shown in Supplementary Movie 1 . Domain switching kinetics In-situ poling results on CSTO using a DF-TEM technique unveil intriguing domain switching kinetics, which can be understood in terms of the creation and annihilation of Z 3 vortex-antivortex (V-VA) pairs. In-situ poling is achieved utilizing fast positive charging [40] , [41] induced by focusing the electron beam ( ∼ 300 nm in diameter) of the TEM at a thin and local area, and the slow reduction of effective electric fields, because of charge dissipation, occurs after removing the focused beam. Thus, in order to observe the in-situ poling process, DF-TEM images are obtained immediately after defocusing the electron beam, before the charges are completely dissipated (on the order of 30 min). 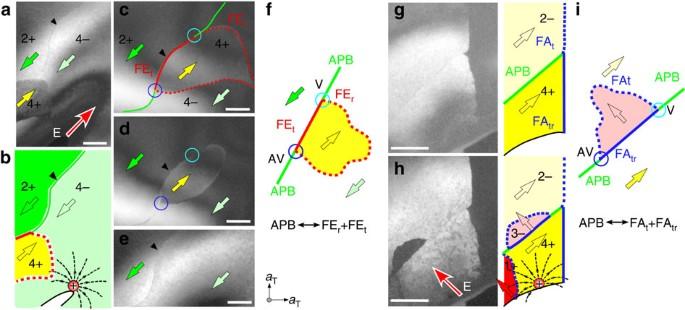Figure 5: The domain switching kinetics under e−beam-induced poling. In-plane DF-TEM images and schematics of domain structures in a CSTO crystal under different directions of induced electric field indicated by red arrows. Coloured arrows and domains represent polarization directions and FE domain states, respectively. Scale bar, 200 nm. (a–e) Image sequences showing a Z3vortex-antivortex (V-AV) pair evolution duringin-situpoling within a single ferroelastic domain. (a,b) The initial state. (c,d) The states during the charge dissipation process after defocusing electron beam. (e) The final state. With a focused electron beam at the sample edge, a direct 180° polarization reversal is observed (4−→4+) via V-AV pair creation (a–c), and the created domain disappears slowly with charge dissipation, which accompanies V-AV pair annihilation (c–e). Cyan and blue circles denote Z3vortices and antivortices, respectively. A black arrowhead is the location marker. (f) Schematic showing the 180° ferroelectric polarization switching via splitting or coalescence of a APB into two ferroelectric walls: APB (green line)→FEt(red-solid)+FEr(red-dotted) DWs. (g,h) Image sequences and schematics showing 90° ferroelectric domain switching near a APB (green line). (g) The initial state. (h) The immediate image after electron beam focused at the sample edge away from the FA boundary (solid blue line). Only 90° poled domains (dark contrast) are observed (2−→3− and 4+→1+). The 90° poled domains are assigned with the rotation order parameter same with those of the initial domains, which is consistent with the low-energy nature of FAtDW. The induced 3− (pink) and 1+ (red) domains return slowly to the initial 2− (light yellow) and 4+ (yellow) states with charge dissipation. (i) Schematic showing a 90° ferroelectric polarization switching within a FA domain via splitting or coalescence of a APB into two ferroelastic walls: APB → FAtr(blue-solid)+FAt(blue-dotted) DWs. Emphasize that there is no hint of the presence of any intermediate states corresponding to 90°polarization reversal during this process. Figure 5a–e shows a Z 3 V-VA pair (cyan and blue circles) within one FA domain behaving coherently with in-situ poling. In-situ poling at a 5 o’clock position near the crystal edge induces a direct 180° polarization reversal of a 4− (light green) domain to a 4+ (yellow) domain ( Fig. 5c ), which is accompanied by the creation of a V-AV pair. The induced 4+ domain shrinks slowly after defocusing the electron beam (from Fig. 5c–e ). Eventually, the induced 4+ domain disappears, and at the same time, the V-AV pair annihilates. This result demonstrates a 180° polarization reversal associated with the creation or annihilation of a Z 3 V-AV pair. Furthermore, the results in Fig. 5a–e reveal that APBs act as nucleation reservoirs for the Z 3 V-AV pair creation and annihilation ( Supplementary Fig. 5 and Supplementary Movie 2 for more details). Figure 5f illustrates that in a Z 3 V-AV pair creation process, a segment of a APB becomes two FE DWs (one FE r DW and the other FE t DW); FE t DWs with a larger energy than that of FE r tend to be pinned at the original APB location, whereas FE r DWs tend to be mobile. This observation is in accordance with the energy hierarchy of FE r ≤FE t ≤APB discussed earlier. Figure 5: The domain switching kinetics under e − beam-induced poling. In-plane DF-TEM images and schematics of domain structures in a CSTO crystal under different directions of induced electric field indicated by red arrows. Coloured arrows and domains represent polarization directions and FE domain states, respectively. Scale bar, 200 nm. ( a – e ) Image sequences showing a Z 3 vortex-antivortex (V-AV) pair evolution during in-situ poling within a single ferroelastic domain. ( a , b ) The initial state. ( c , d ) The states during the charge dissipation process after defocusing electron beam. ( e ) The final state. With a focused electron beam at the sample edge, a direct 180° polarization reversal is observed (4−→4+) via V-AV pair creation ( a – c ), and the created domain disappears slowly with charge dissipation, which accompanies V-AV pair annihilation ( c – e ). Cyan and blue circles denote Z 3 vortices and antivortices, respectively. A black arrowhead is the location marker. ( f ) Schematic showing the 180° ferroelectric polarization switching via splitting or coalescence of a APB into two ferroelectric walls: APB (green line)→FE t (red-solid)+FE r (red-dotted) DWs. ( g , h ) Image sequences and schematics showing 90° ferroelectric domain switching near a APB (green line). ( g ) The initial state. ( h ) The immediate image after electron beam focused at the sample edge away from the FA boundary (solid blue line). Only 90° poled domains (dark contrast) are observed (2−→3− and 4+→1+). The 90° poled domains are assigned with the rotation order parameter same with those of the initial domains, which is consistent with the low-energy nature of FA t DW. The induced 3− (pink) and 1+ (red) domains return slowly to the initial 2− (light yellow) and 4+ (yellow) states with charge dissipation. ( i ) Schematic showing a 90° ferroelectric polarization switching within a FA domain via splitting or coalescence of a APB into two ferroelastic walls: APB → FA tr (blue-solid)+FA t (blue-dotted) DWs. Emphasize that there is no hint of the presence of any intermediate states corresponding to 90°polarization reversal during this process. Full size image We also studied electron beam-induced poling in different directions. The switching process depends significantly on the electric field orientation ( Supplementary Fig. 5 ). For example, Fig. 5g shows another region with two antiphase 4+ (yellow) and 2− (light yellow) domains with slightly different bright contrasts located next to an APB (green line). Interestingly, when the electron beam is focused on the specimen edge away from FA DWs (blue lines) and an electric field (red/white arrow in Fig. 5h ) perpendicular to the original polar axis is induced, a 90° polarization switching from a bright 2− (light yellow) to dark 3− (pink) triangular domain is observed. The induced 3− domain returns slowly to the initial 2− state with charge dissipation. This process is involved with the splitting or coalescence of an APB to two FA DWs; one FA tr DW and the other FA t DW ( Fig. 5i ). The created FA tr DW with high energy stays at the original APB location, whereas the created FA t DW with low energy tends to be mobile. We observe a direct 180° (90°) polarization switching, instead of going through an intermediate 90° (180°) polarization state in the in-situ poling process. We emphasize that the coherent DW network of Z 4 × Z 2 domains with Z 3 vortices and some highly curved walls ( Fig. 3 ) leads to the presence of charged DWs and APBs. The presence of Z 3 -vortices instead of the formation of antiparallel domains separated by neutral walls also indicates that a moderate energy difference among five types of DWs. In particular, those APBs serve as primary nucleation centres for 180° and 90° polarization switching, and the presence of mobile n -type charge carriers, screening the polar discontinuity at charged DWs, are responsible for the large conduction of head-to-head DWs [3] . Note that the APBs with the discontinuity of both octahedral tilting (t) and rotation (r) costs more energy and one ABB splits into two FE/FA walls under an external electric field, so an APB becomes a nucleation centre of a new poled domain ( Fig. 5 ). This can also happen in high-energy FA tr DWs as shown in the Fig. 6 . This zipper-like splitting of high-energy DWs accompanies the emergence of Z 3 V-AV pairs. The high-energy APB and FA tr DWs dominate the nucleation controlled kinetics of polarization flipping, while the low-energy FE r and FA t DWs tend to move steadily with an external electric field, which can be responsible for the DWs motion kinetics. Emphasize that unlike expected minor roles of APBs with just translation phase shift, APBs dominate the FE polarization switching in hybrid improper FE (Ca,Sr) 3 Ti 2 O 7 . These unexpected discoveries of the role of APBs and the domain topology relevant to the presentence of abundant conducting DWs should be further investigated for deeper understanding and nano-engineering of the domains and DWs in hybrid improper FEs. 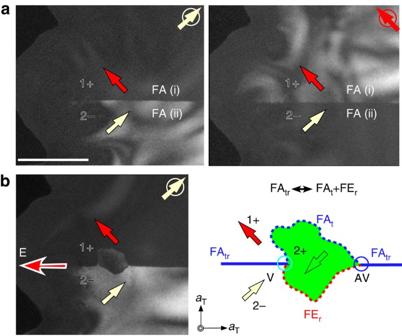Figure 6: Domain switching kinetics in the absence of APBs in CSTO. (a) In-plane DF-TEM images show two ferroelastic (FA(i) and FA(ii)) regions. Domain states 2− (light yellow arrow) and 1+ (red arrow) are assigned based on diffraction patterns and the assumption of a non-charged head-to-tail wall. (b) Polarization domain evolutions across a FAtrboundary. Election beam focused at the end of a FA boundary close to the sample edge induces an electric field indicated by a red/white arrow. A polarization switching (dark grey contrast) from 1+ → 2+ in FA(i) and 2−→2+ in FA(ii) is observed. The right-side cartoon shows a schematic of the domain switching via a splitting/merging of FAtr→ FAt+FErDWs. A high energy FAtrDW becomes two DWs with lower energies; one ferroelectric FErDW and the other ferroelastic FAtDW, which is consistent with our energy hierarchy. Both FAtand FErDWs tend to be mobile and highly curved, which is again consistent the low energy nature of FAtand FErDWs in our energy hierarchy. Cyan and blue circles denote Z3vortex (V) and antivortex (AV), respectively. Scale bar, 500 nm. Figure 6: Domain switching kinetics in the absence of APBs in CSTO. ( a ) In-plane DF-TEM images show two ferroelastic (FA(i) and FA(ii)) regions. Domain states 2− (light yellow arrow) and 1+ (red arrow) are assigned based on diffraction patterns and the assumption of a non-charged head-to-tail wall. ( b ) Polarization domain evolutions across a FA tr boundary. Election beam focused at the end of a FA boundary close to the sample edge induces an electric field indicated by a red/white arrow. A polarization switching (dark grey contrast) from 1+ → 2+ in FA(i) and 2−→2+ in FA(ii) is observed. The right-side cartoon shows a schematic of the domain switching via a splitting/merging of FA tr → FA t +FE r DWs. A high energy FA tr DW becomes two DWs with lower energies; one ferroelectric FE r DW and the other ferroelastic FA t DW, which is consistent with our energy hierarchy. Both FA t and FE r DWs tend to be mobile and highly curved, which is again consistent the low energy nature of FA t and FE r DWs in our energy hierarchy. Cyan and blue circles denote Z 3 vortex (V) and antivortex (AV), respectively. Scale bar, 500 nm. Full size image Sample preparation Single-crystalline CSTO and CMTO were grown by using optical floating zone methods. For polycrystalline Ca 3-x Sr x Ti 2 O 7 (Ca 3 Mn 2-x Ti x O 7 ) feed rods, stoichiometric CaCO 3 , SrCO 3 and TiO 2 (MnO 2 ) were mixed, ground, pelletized and sintered at 1,350–1,550 °C for 30 h. Substituting Sr into the Ca site in Ca 3 Ti 2 O 7 induces the reduced size of FA domains suitable for TEM studies. It was very difficult to grow high-quality single crystals of pure Ca 3 Mn 2 O 7 , but the slight substitution of Ti into the Mn site of Ca 3 Mn 2 O 7 stabilizes crystal growth without changing the relevant physics of Ca 3 Mn 2 O 7 . Crystals are highly cleavable, and were cleaved in air for optical microscopy observation. Transparent amber coloured CSTO single crystals and non-transparent dark blue coloured CMTO present a similar polar orthorhombic symmetry (space group #36, A2 1 am ) [3] , [30] , [33] . Crystal structure and lattice parameters were examined by X-ray diffraction with a Philips XPert powder diffractometer and the general structure analysis system program. CMTO possesses a one and half larger FA distortion (that is, orthorhombicity defined by ( a − b )/( a + b )*100%, ∼ 0.08 %) than Ca 3 Ti 2 O 7 ( ∼ 0.05 %). Cycling the CMTO sample temperature through Tc leads to a completely different irregular FA pattern, indicating that the domain formation is not simply due to pinning by disorder such as chemical defects or dislocations. Dark-field TEM measurement Specimens for DF-TEM studies were fabricated on Ca 3 Ti 2 O 7 (CTO), Ca 2.55 Sr 0.45 Ti 2 O 7 (CSTO) and Ca 3 Mn 1.9 Ti 0.1 O 7 (CMTO) single crystals ( ∼ 1 × 2 × 0.1 mm 3 in size) by mechanical polishing, followed by Ar-ion milling and studied using a JEOL-2010F TEM. Note that one TEM specimen can include up-to-a-hundred FA domains for observations, and we have examined two CSTO, one CTO and two CMTO TEM specimens. Although the width of FA domains varies, our conclusion on the Z 4 × Z 2 domain structure with Z 3 vortex patterns and five types of DWs is universal in all specimens that we have observed. We also found that the FA domain size depends little on various heat treatment conditions in both CSTO and CMTO. We observed vortex domains by DF-TEM imaging taking two diffraction vectors: (i) superlattice g 1 ± =±3/2(1, 1, 0) T =±(3, 0, 0) orth spots, parallel to the polar axis in [001] T zone and (ii) superlattice g 2 ± =±3/2(−1, 1, 2) T =±(0, −3, 3) orth spots, perpendicular to the polar axis in [1, −1, 1] T zone, 15° tilting from c -axis. 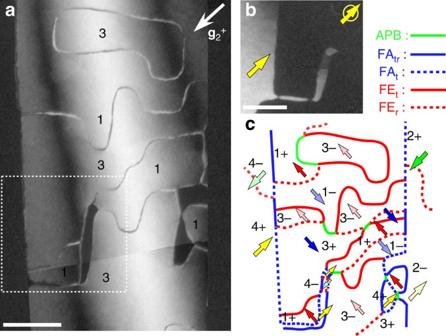Figure 7: A full assignment of domain states and wall types in CSTO. (a) A 2 × 2.9 μm2mosaic of DF-TEM images were taken using the superlatticeg2+=3/2(−1, 1, 2)Tspot of domain FA(i) in a CSTO crystal along [1–11]T, showing only part of DWs in this condition. Neither domain contrast nor curved and broad FErDWs can be visualized under this condition. A tilting (1stor 3rdquadrants) configuration are depicted. Scale bar, 500 nm. (b) A DF-TEM image taken using another superlatticeg1+spot (yellow circle), 90° relative to the one for FA(i), within the white rectangular box. The bright contrast corresponds to the other four types of 180° FE domains (2+, 2−, 4+ and 4−) inside the FA(ii) region. (c) A schematic domain and domain wall configuration for the area ina, including various FE domains and five types of DWs. Figure 7a shows DF-TEM images taken at the same area as Fig. 3a using the superlattice g 2 + spot. Non-FE structural boundaries can be visualized under this condition as the g 2 + vector is perpendicular to the polar a orth -axis and the FE contribution is minimized. To avoid confusion with APBs, those boundaries observed in this condition without considering the polarization effect are named as ‘B-boundaries’. The appearance of ‘B-boundaries’ is a result of symmetry breaking through the tetragonal-to-orthorhombic phase transition. They tend to show step-like features along the <100> T direction. Based on the domain switching kinetics shown in Fig. 5 , we argue that those ‘B-boundaries’ are either APBs or FE t DWs, so APBs and FE t DWs tend to be <100> T -oriented. Contrarily, FE r DWs show wavy features with no preferred orientation, because of the so-called ‘rotational compatibility conditions’ [38] . The role of ‘B-boundaries’ is further discussed in Supplementary Fig. 5 . Figure 7b shows DF-TEM image taken using the superlattice g 1 + spot, showing the domain contrast of neighbouring FA(ii) region. A full assignment of domain states and DW types in a CSTO crystal is shown in Fig. 7c based on the domain contrast shown in Figs 3a and 7b and wall features associated with local distortions discussed below. Figure 7: A full assignment of domain states and wall types in CSTO. ( a ) A 2 × 2.9 μm 2 mosaic of DF-TEM images were taken using the superlattice g 2 + =3/2(−1, 1, 2) T spot of domain FA(i) in a CSTO crystal along [1–11] T , showing only part of DWs in this condition. Neither domain contrast nor curved and broad FE r DWs can be visualized under this condition. A tilting (1 st or 3 rd quadrants) configuration are depicted. Scale bar, 500 nm. ( b ) A DF-TEM image taken using another superlattice g 1 + spot (yellow circle), 90° relative to the one for FA(i), within the white rectangular box. The bright contrast corresponds to the other four types of 180° FE domains (2+, 2−, 4+ and 4−) inside the FA(ii) region. ( c ) A schematic domain and domain wall configuration for the area in a , including various FE domains and five types of DWs. Full size image Local structural distortions at FE and FA DWs Supplementary Fig. 2a shows a (110) T -oriented FE t DW between two neighbouring 1+ and 3+ domains, where the octahedral tilting ( a − a − c 0 ) may be fully suppressed if octahedral tilting changes across the DW by passing through the tetragonal central position ( Supplementary Fig. 3 ). On the other hand, Supplementary Fig. 2b shows a FE r DW between neighbouring 1+ and 1− domains, where neither of the two lattice modes becomes zero. Thus, FE r DW may accompany a lower energy than FE t DW does ( Supplementary Fig. 3 ). Given that the oxygen octahedra in A 3 B 2 O 7 are connected by sharing the oxygen atom in their corner, at those DWs, some shift of equatorial oxygens (indicated by red spheres in black circles in Supplementary Fig. 2a,b ) that locate between Ti sites (cyan spheres) is expected. Enlarged views of the octahedra across the DWs ( Supplementary Fig. 2a,b upper panels) clearly show a larger octahedral mismatch at the FE r DW than that at the FE t DW when observed along the [100] T axis. Experimentally, APBs can be identified from the domain contrast without ambiguity ( Fig. 2b–d ). Although DWs can deviate from typical orientations to minimize the wall energy in the thin foil-type geometry of TEM specimens, we constantly observe a narrow sharp-contrast wall and a relatively broad wall with clear interference fringes near a Z 3 vortex core. As strain provides the main diffraction contrast change in our DF-TEM images, we associate the narrow sharp-contrast lines with a less octahedral mismatch to FE t DWs in the ab -plane projection. This is, indeed, the case for a sharper wall between domain i and iii shown in Fig. 2d and between domains 1− and 3− or domains 1+ and 3+ shown in Fig. 4d,e , which we therefore assign as FE t DWs. A clear interference fringes or wavy features can be observed between domains ii and iii ( Fig. 2d ) and domains 1− and 1+ or domains 3− and 3+ ( Fig. 4d,e ), suggesting an inclined nature and a strong strain gradient as expected in FE r DWs. Phase-field modeling To describe the distortion relative to the high symmetry phase with space group I4/mmm , three sets of order parameters are used, that is, ϕ i ( i =3) for the oxygen octahedral rotation around the x 3 axis, and θ i ( i =1,2) and P i ( i =1,2) for the octahedral tilt and polarization component along the x i ( i =1,2) pseudocubic axis, respectively [23] , [42] . The total free energy density can be expressed by where α ij , α ijkl , β ij , β ijkl , t ijkl , d and γ ij are the coefficients of Landau polynomial, κ ijkl , δ ijkl and g ijkl are gradient energy coefficients, c ijkl is the elastic stiffness tensor, ɛ ij and are the total strain and eigen strain, and E i is the electric field given by E i =− ϕ , i with ϕ the electrostatic potential. Note that γ ij>0 , and the term dϕ 3 ( θ 1 P 1 + θ 2 P 2 ) determines that ( P 1 , P 2 ,0) and ( θ 1 , θ 2 ,0) are parallel or antiparallel, dependent on the sign of ϕ 3 . The eigen strain is related to the order parameters through , where λ ijkl and h ijkl are coupling coefficients. Here the coupling between polarization and strain is ignored, as the secondary order parameter polarization is always parallel or antiparallel to the octahedral tilt order parameter. The Landau polynomial is expanded based on group theory analysis [42] , and the related coefficients are obtained by first-principles calculations [38] , [43] , [44] , [45] , [46] , [47] , [48] ( Tables 1 , 2 , 3 ). Anisotropic properties are assumed in gradient energy coefficients κ ijkl and δ ijkl , that is, κ iiii κ ijij , δ iiii δ ijij (ref. 38 ). The phase-field equations are solved with the initial condition of zero plus a small random noise for the order parameter components [49] . Periodic boundary conditions are employed along the three directions. The system size is 1,024Δ x × 1,024Δ x × 1Δ x , and the grid spacing is Δ x= 0.30 nm. Coefficients of Ca 3 Ti 2 O 7 used in the phase-field simulations Total energy calculations based on density functional theory within the generalized-gradient approximation given by the revised Perdew–Becke–Erzenhof parameterization for solids [43] using the projector augmented wave method [44] , [45] implemented in the Vienna Ab initio Simulation Package [46] , [47] are used to obtain the coefficients found in the Landau polynomial (Methods, Equation (1)). A plane-wave cutoff of 600 eV and a 4 × 4 × 1 k -point mesh with Gaussian smearing (0.10 eV width) is used for the Brillouin-zone integrations. The calcium 3 s , 3 p and 4 s electrons, Ti 3 p , 3 d and 4 s electrons, and O 2 s and 2 p electrons are treated as valence states. The coefficients for the Landau polynomial are obtained by fitting the calculated total energies as a function of magnitude of the order parameters for the configurations corresponding to displacement patterns for each individual mode or combination of modes. The values for the relevant coefficients are given in Table 1 . In all total energy calculations, the lattice constants are fixed at the calculated equilibrium values for the high-symmetry I4/mmm structure (parent clamping approximation). The total elastic stiffness tensor, including the contributions for distortions with rigid ions and the contributions from relaxed ions, is also obtained by calculating the strain–stress relations [48] in the I4/mmm structure ( Table 2 ). The gradient energy coefficients κ ijkl , δ ijkl and g ijkl are estimated based on the gradient energy coefficients of BiFeO 3 (ref. 38 ) as both the two systems show the coexistence of oxygen octahedral tilt and polarization, and are listed in Table 3 . Note that the domain structures are determined by the relative magnitude of different gradient energy coefficients, and will be hardly affected by the specific values. Data availability The authors declare that all source data supporting the findings of this study are available within the article and the Supplementary Information File . How to cite this article: Huang, F.-T. et al . Domain topology and domain switching kinetics in a hybrid improper ferroelectric. Nat. Commun. 7:11602 doi: 10.1038/ncomms11602 (2016).